Targeting QKI-7 in vivo restores endothelial cell function in diabetes Vascular endothelial cell (EC) dysfunction plays a key role in diabetic complications. This study discovers significant upregulation of Quaking-7 (QKI-7) in iPS cell-derived ECs when exposed to hyperglycemia, and in human iPS-ECs from diabetic patients. QKI-7 is also highly expressed in human coronary arterial ECs from diabetic donors, and on blood vessels from diabetic critical limb ischemia patients undergoing a lower-limb amputation. QKI-7 expression is tightly controlled by RNA splicing factors CUG-BP and hnRNPM through direct binding. QKI-7 upregulation is correlated with disrupted cell barrier, compromised angiogenesis and enhanced monocyte adhesion. RNA immunoprecipitation (RIP) and mRNA-decay assays reveal that QKI-7 binds and promotes mRNA degradation of downstream targets CD144, Neuroligin 1 (NLGN1), and TNF-α-stimulated gene/protein 6 (TSG-6). When hindlimb ischemia is induced in diabetic mice and QKI-7 is knocked-down in vivo in ECs, reperfusion and blood flow recovery are markedly promoted. Manipulation of QKI-7 represents a promising strategy for the treatment of diabetic vascular complications. To date, there are over 400 million people with diabetes worldwide and the prevalence of the disease is predicted to continue to rise [1] , [2] . Macrovascular (coronary artery disease, stroke, and peripheral artery diseases) and microvascular (retinopathy, nephropathy, and neuropathy) complications are the main drivers for the morbidity and mortality related to diabetes [3] , [4] . Patients with diabetes are known to have a two- to fourfold increased risk of cardiovascular diseases [4] , [5] , [6] . Vascular endothelial cells (ECs) are critical for the maintenance of vessel integrity as well as regulation of angiogenesis, inflammatory infiltration, monocyte adhesion, platelet aggregation, and intercellular barrier [7] , [8] . Under diabetic conditions, vascular complications are initiated by EC dysfunction leading to abnormal angiogenesis, enhanced permeability, increased monocyte adhesion and a trend toward increased thrombogenesis and blood flow impairment [5] . Extensive evidence from clinical studies and diabetic animal models revealed the increase of reactive oxygen species (ROS), downregulation of nitric oxide synthase (eNOS), and attenuated nitric oxide (NO) levels in vascular ECs, as important mechanisms underlying the pathogenesis of EC dysfunction [9] . These implicate the involvement of a number of signaling pathways such as PKC, PI3K/AKT, MAPK, NF-kB, and Rho/ROCK amongst others [10] , [11] , [12] . Hence, therapeutic strategies to restore NO levels and suppress oxidative stress hold promise to restore EC function. However, it is still very challenging to rescue diabetic EC dysfunction. A comprehensive understanding of the mechanisms underlying dysfunction of ECs in diabetes is critical to the development of more effective treatments of vascular complications. The advent of induced pluripotent stem cell (iPSC) reprogramming technology has made it possible to generate disease models from patient somatic cells [13] , [14] . Using well-established protocols, iPSCs can be efficiently differentiated into ECs. Diabetic patient-derived iPS-ECs thereby provide a valuable cell model for the study of diabetic EC pathophysiology and drug screening with direct clinical relevance. Diabetes leads to dramatic alteration of gene expression profiles in ECs, including genes related to angiogenesis, inflammation, and cell adhesion [15] , [16] , with transcriptional and post-transcriptional regulation systems cooperating to finely regulate gene expression in vascular ECs. RNA-binding proteins (RBPs) play critical roles in post-transcriptional regulation through formation of ribonucleoprotein (RNP) complexes with specific RNA sequences and/or RNA structures. Recent studies have implicated RBP dysregulation in diabetic complications [17] , [18] . Quaking (QKI) is one of the RBPs related to diabetic cardiomyopathy and atherosclerosis. QKI belongs to the signal transduction and activation of RNA (STAR) family, featuring conserved SH2, SH3, and KH RNA-binding domains and participates in the regulation of pre-mRNA splicing, mRNA nuclear exportation, mRNA stability, protein translation, and signal transduction [19] . Three of the central QKI transcript isoforms named QKI-5 , QKI-6 , and QKI-7 share identical sequences in most of their coding districts but differ at the very end of the C-terminus. All three QKI isoforms are expressed in vascular ECs, with QKI-5 being the most abundant [20] . QKI-5 knockout mice are embryonic lethal at E10-12.5 due to disrupted vascular development along with decreased PECAM-1 and Tie-2 expression [21] . Recent work in our group demonstrated that QKI-5 significantly promoted angiogenesis and enhanced blood flow recovery in experimental hindlimb ischemia. Direct binding of QKI-5 to the 3′UTR and stabilization of STAT3 mRNA was verified, which in turn stabilized VE-cadherin and activated VEGFR2 [22] . We have also recently shown that QKI-6 promotes HDAC7 splicing and benefit vascular smooth muscle cell (VSMCs) induction from iPSCs. QKI-6 overexpressing VSMCs in combination with QKI-5 overexpressing ECs significantly enhanced the formation of vascular structures with in vivo Matrigel assay, corroborating their roles to support angiogenesis [23] . While both QKI-5 and QKI-6 contribute positively to angiogenesis, they act in various ways in different cell types, indicating the key impacts of the unique C-terminus sequences on their functions. The third QKI isoform QKI-7 also has a specific C-terminus and its function concerning angiogenesis is still unknown. Different to the C-tail nuclear localization signal with QKI-5, QKI-7 C-terminal sequence is weakly related to SH3 domain, suggesting a different subcellular localization. In this study, QKI-7 shows predominantly cytoplasmic localization indicating that its function may not be directly involved in RNA splicing. We have discovered that QKI-7 is significantly upregulated in mouse iPSC-derived ECs (miPS-ECs) treated with high glucose and human iPS-ECs from diabetic patients. QKI-7 is also found to be highly expressed in human coronary arterial ECs isolated from diabetic donors, and on blood vessels obtained from diabetic critical limb ischemia patients undergoing a lower-limb amputation. QKI-7 binds and promotes mRNA degradation of downstream targets CD144, NLGN1, TSG6 and contributes to vascular EC dysfunction. This has set up the hypothesis that QKI-7 holds a key role in the pathogenesis of diabetic EC dysfunction. Importantly, in this study we present robust evidence that targeting QKI-7 in vivo restores EC function in diabetes based on fully-defined mechanisms, presenting a potential therapeutic route for the treatment of diabetic vascular complications. Mouse iPSC (miPSC) differentiation toward endothelial cells miPSCs were seeded on collagen IV-coated culture dishes and differentiated toward vascular ECs cultured in differentiation media (α-MEM + 10% FBS) supplemented with 25 ng/ml vascular endothelial growth factor (VEGF) for 2–10 days. The differentiated cells adopted a typical cobblestone-like EC morphology (Supplementary Fig. 1A ). To verify the identity of miPSC-derived ECs (miPS-ECs), the expression of EC markers was investigated, demonstrating that CD144 and FLK1 increased in a time-dependent manner (Supplementary Fig. 1B ). The protein expression of EC markers, CD144, FLK1, and eNOS was confirmed by western blots (Supplementary Fig. 1C ). At day 6 of differentiation, flow cytometry demonstrated that 78% of cells were CD144/VE-Cadherin positive, indicating the high efficiency of EC induction from miPSCs (Supplementary Fig. 1D , Supplementary Fig. 12 ). By immunofluorescence confocal microscopy, considerable expression of CD144 and ZO-1 was observed at cell–cell junctions, a classic feature of vascular ECs (Supplementary Fig. 1E ). When seeded on top of solidified Matrigel beds, miPS-ECs readily formed tube-like structures indicating their functional capacity (Supplementary Fig. 1F ). These results show that miPSCs were efficiently differentiated into functional vascular ECs. QKI-7 is inversely regulated by the factors CUG-BP and hnRNPM When treated with high glucose, miPS-ECs showed dose-dependent elevation of QKI-7 gene expression, corroborated at protein level by western blot (Fig. 1a, b ). However, the expression level of the other QKI isoforms, QKI-5 and QKI-6 , was not affected (Supplementary Fig. 2A, B ). Notably, QKI-7 shares the same N-terminal sequence with the other isoforms but differs only at the last exon due to alternative splicing. Therefore, a specific alternative splicing mechanism may be involved in the upregulation of QKI-7 by high-glucose treatment. Fig. 1: QKI-7 dynamics under high glucose related to CUG-BP and hnRNPM. Upon high-glucose treatment of miPS-ECs, QKI-7 expression showed a dose-dependent increase at both mRNA ( p values: 0.023, 0.013, 0.0034, 0.0016, and <0.0001) and protein levels ( a , b ). CUG-BP was upregulated by high-glucose treatment dose-dependently ( p values: 0.013, 0.0032, 0.0004) ( c ). hnRNPM expression was downregulated by high-glucose treatment ( p values: 0.0064, 0.001, 0.0069) ( d ). CUG-BP overexpression enhanced QKI-7 expression ( p value: 0.0012) ( e ). hnRNPM overexpression suppressed QKI-7 expression ( p value: 0.0011) ( f ). QKI-7 upregulation by overexpressed CUG-BP and downregulation by ectopic hnRNPM is shown by western blot ( g ) and quantified in ( h ) ( p values: 0.0021, 0.0099). L-glucose-treated cells have been used as controls in these experiments. Data are from three biologically independent experiments. Error bars represent mean ± SEM ( n = 3). P values are shown: * p < 0.05, ** p < 0.01, *** p < 0.001, **** p < 0.0001 (two-tailed t test). The source data are provided as a Source data file. Full size image In search of QKI-7 regulators under high-glucose conditions, 35 predicted binding splicing factors to QKI-7 were examined for changes in their expression profiles. Two of these splicing factors showed dynamic changes in response to glucose treatment: CUG-BP was upregulated by high glucose in a dose-dependent manner consistent with QKI-7 level alteration, while hnRNPM expression decreased under high-glucose treatment (Fig. 1c, d ). We supposed that CUG-BP and hnRNPM were antagonistic with respect to QKI-7 regulation and examined their impact on QKI-7 expression. Indeed, when CUG-BP was overexpressed in miPS-ECs, QKI-7 expression was upregulated, while ectopic expression of hnRNPM decreased QKI-7 levels (Fig. 1e, f ). In line with their effects on QKI-7 gene expression, overexpression of either CUG-BP or hnRNPM had opposing effects on QKI-7 protein expression in miPS-ECs (Fig. 1g, h ). A specific alternative splicing of exon 7 in the QKI gene generates the QKI-7 isoform [24] . According to the conserved RNA binding motifs of CUG-BP and hnRNPM ( http://rbpmap.technion.ac.il/ ), there are a number of predicted binding sites for the two RNA splicing factors within the QKI-7 gene sequence within intron 6 and intron 6–exon 7 interface districts (Supplementary Fig. 3 ). This suggests that direct binding of CUG-BP and hnRNPM to this region promotes or inhibits the generation of QKI-7 transcript through alternative splicing regulation. Notably, further experiments confirmed the binding of CUG-BP and hnRNPM to these QKI-7 gene regions by RNA immunoprecipitation (RIP) assays. These data are shown in Supplementary Fig. 3A, B , respectively. Therefore, the CUG-BP and hnRNPM splicing factors regulate QKI-7 levels diametrically to maintain homeostasis by direct binding. Under diabetic conditions, this balance appears to become disrupted due to dysregulation of CUG-BP and hnRNPM leading to QKI-7 upregulation. Interestingly, neither the QKI-7 nor the splicing factors hnRNPM and CUG-BP expression levels altered when human Fibroblasts were treated with high glucose over a period of 3 and 6 days (Supplementary Figure 4A, B ). L-glucose-treated cells were used as controls in these experiments. These findings demonstrate a specific role of QKI-7 in ECs upon high-glucose conditions. 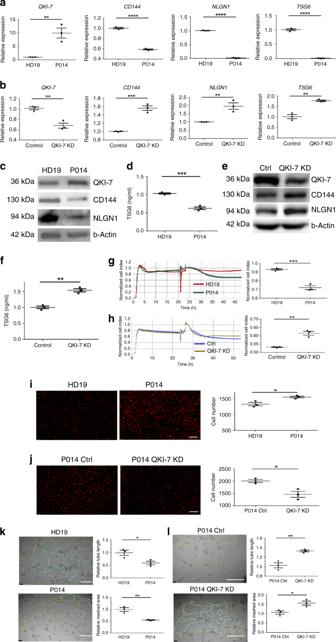Fig. 4: QKI-7 in diabetic iPS-ECs was correlated with EC dysfunction. Compared with the non-diabetic iPS-EC HD19 control, iPS-EC P014 derived from a patient with diabetes showed significantly higher level of QKI-7 (pvalue: 0.0083) accompanying decreased expression of CD144, NLGN1, and TSG6 (pvalues: <0.0001) (a). When QKI-7 was knocked down (pvalue: 0.0042), iPS-ECs showed increased expression of CD144, NLGN1, and TSG6 (pvalues: 0.0006, 0.0081, 0.0019) (b). Comparison of protein level between diabetic iPS-EC P014 and non-diabetic HD19 was shown by western blot (c) and ELISA (pvalue: 0.0005) (d). Upon QKI-7 knockdown, western blot showed increase of CD144 and NLGN1 (e) and ELISA verified the upregulation of TSG6 (pvalue: 0.0011) (f). Diabetic iPS-EC P014 showed significantly lower RTCA cell index than non-diabetic HD19 indicating a permeability increase (pvalue: 0.0009) (g). When QKI-7 was knocked down, P014 RTCA cell index was enhanced, showing the alleviation of cell barrier defect (pvalue: 0.0019) (h). Compared with the non-diabetic HD19, the diabetic iPS-EC P014 displayed more THP-1 monocyte adhesion (pvalue: 0.0203) (i) which was ameliorated by QKI-7 knockdown (pvalue: 0.0163) (j). In tube formation assay, diabetic iPS-EC P014 formed less capillary structure than non-diabetic HD19 cells, measured by shorter tube branch length and smaller meshed area (pvalues: 0.0312, 0.0052) (k) which was reversed by QKI-7 knockdown (pvalues: 0.0061, 0.0225) (l), the data were normalized by setting the control group as 1. Scale bari,j: 100 μm; scale bark,l: 200 μm. Data are from three biologically independent experiments. Error bars represent mean ± SEM (n= 3).Pvalues are shown: *p< 0.05, **p< 0.01, ***p< 0.001, ****p< 0.0001 (two-tailedttest). Source data are provided as a Source data file. QKI-7 impacts on critical genes and disrupts EC function The induction of QKI-7 by high-glucose treatment indicates a potentially important role in the pathogenesis of diabetes. To validate this hypothesis, QKI-7 was overexpressed in miPS-ECs to investigate its direct effects on the expression level of genes involved in EC function (Fig. 2a ). All the QKI isoforms have the same conserved RNA binding domain. André Galarneau and Stephane Richard defined the QKI response element (QRE) bipartite consensus sequence and predicted 1430 QKI RNA-binding targets [25] . To explore the QKI-7 RNA targets, 35 EC function-related genes from this published candidate list were screened. When QKI-7 was overexpressed in miPS-ECs, 3 genes of the 35 candidates were found to be downregulated, including CD144 , TSG6 , and NLGN1 (Fig. 2b ). Western blot confirmed the decrease of CD144 and NLGN1 at protein level (Fig. 2c ) and TSG6 downregulation was verified by ELISA (Fig. 2d ). CD144 is a major component of EC adherens junctions which is critical for EC barrier function and angiogenesis [26] . TSG6 is a TNF-α-inducible, secretory hyaluronic acid-binding protein that acts as a regulator of cell–cell and cell–matrix interactions as well as a potent anti-inflammatory factor [27] , [28] . NLGN1 collaborates with α6 integrin to direct the interaction of ECs with the underlying extracellular matrix during vascular development. According to the functional characteristics of CD144, NLGN1, and TSG6, the increased QKI-7 under high glucose may disrupt EC functions, such as cell barrier formation, angiogenesis, and monocyte adhesion through downregulation of these three genes. These EC functions were therefore tested in miPS-ECs following QKI-7 overexpression. Cell barrier properties of iPS-ECs were investigated using the real-time cell analysis (RTCA) with the xCELLigence system. This method measures cell adhesion using high-density gold electrode arrays in a non-invasive, label-free manner. The iPS-ECs were cultured on the E-Plate with gold electrodes on the bottom of wells which are responsible for the completion of electric circuit of the applied electric potential. The impedance reflected the cell–cell interaction of adherent cells. The RTCA software converted impedance values into the Cell Index (CI), which serves as a readout of cell adhesion. In this study, QKI-7 -overexpressing iPS-ECs showed decreased CI by xCelligence assay after VEGF-induced EC barrier disruption compared with control cells (ECs overexpressing an empty vector), indicating the defective cell barrier function associated with QKI-7 high expression (Fig. 2e ). In the Matrigel tube formation assay, fewer tube-like structures were quantified and significantly shorter inter-connecting branches with an overall smaller meshed area was observed in iPS-ECs overexpressing QKI-7 compared with controls, demonstrating an impaired angiogenic capacity (Fig. 2f ). In the pathogenesis of diabetes, one of the earliest events in inflammation and atherosclerosis is increased adhesion of monocytes to the activated vascular ECs [29] . When co-cultured with Vybrant-labeled THP-1 monocytes, QKI-7 overexpressing ECs adhered to greater numbers of THP-1 cells compared with controls ECs (Fig. 2g ). This suggests that QKI-7 upregulation may contribute to enhanced monocyte adhesion and subsequently altered blood perfusion which in turn will influence vessel function and structure, inflammatory cell infiltration, and development of atherosclerosis in diabetes. The downregulation of anti-inflammatory factor TSG6 by QKI-7 may be at least partly responsible for these events. In addition to the decrease of TSG6 , it was found that QKI-7 overexpression led to a substantial induction of IL-1β (Supplementary Fig. 5A ). Moreover, QKI-7 knockdown by siRNA reduced IL-1β (Supplementary Fig. 5B ), while IL-1β was highly expressed on human iPS-ECs generating from diabetic donors (Supplementary Fig. 5C ). These findings suggest that QKI-7 has a significant influence on inflammatory pathways in diabetes through regulation of multiple factors. Fig. 2: QKI-7 affected genes/proteins expression and EC functions. QKI-7 overexpression ( p value: 0.0006) in miPS-ECs led to downregulation of EC function-related genes CD144, TSG6, and NLGN1 ( p values: 0.0027, 0.0012, 0.0014) ( a , b ). Protein level alteration of QKI-7 and target candidates was verified by western blot from three independent experiments ( c ) and ELISA ( p value: 0.0038) ( d ). QKI-7 overexpressing miPS-ECs showed decreased cell index with xCELLigence real-time cell analysis (RTCA) indicating disrupted cell barrier and increased permeability ( p value: 0.0073) ( e ). In tube formation assay, QKI-7 overexpressing miPS-ECs formed less capillary structure than control cells, measured by shorter tube branch length and smaller meshed area ( p values: 0.0069, 0.0024) ( f ). QKI-7 overexpression enhanced THP-1 adhesion to miPS-ECs ( p value: 0.0107) ( g ), the data were normalized by setting the control group as 1. Data are from three biologically independent experiments. Error bars represent mean ± SEM ( n = 3), * p < 0.05, ** p < 0.01, *** p < 0.001 (two-tailed t test). The source data are provided as a Source data file. Full size image QKI-7 correlates with EC dysfunction in human diabetic ECs To study the role of QKI-7 in diabetic EC dysfunction, human iPSCs (hiPSCs) were generated from blood samples of people with diabetes, age, and sex-matched non-diabetic donors, and differentiated into vascular ECs, using a fast and highly efficient approach that we have recently reported [30] . Those hiPS-ECs assumed a typical cobblestone monolayer morphology (Fig. 3a ). After MACS selection using CD144-conjugated magnetic beads, a pure EC population was obtained as shown by FACS analysis (Fig. 3b , Supplementary Fig. 12 ). The iPS-ECs displayed strong expression of EC-specific markers CD31, CD144, KDR, and eNOS (Fig. 3d ). Immunocytochemistry confirmed the expression of CD31, CD144, and ZO-1 as well as their localization at cell–cell junctions (Fig. 3c ). Of note, QKI-7 showed perinuclear cytoplasmic localization which is consistent with previous reports [31] . RNA splicing occurs in the nucleus either during or immediately after the transcription process; therefore, QKI-7’s cytoplasmic location suggests that its primary function may not be to regulate RNA splicing. Like miPS-ECs, when seeded on solidified, reduced growth factor Matrigel, hiPS-ECs formed capillary-like structures showing their functional characteristics (Fig. 3e ). Fig. 3: Human iPS cells differentiation toward ECs. Morphology of hiPSCs and their EC differentiated counterparts are shown by bright field microscopy. Scale bar: 50 μm ( a ). Flow cytometry showed the pure population of hiPS-derived ECs after MACS selection using CD144 magnetic beads ( b ). Immunofluorescence confocal image showing that the differentiated ECs expressed the EC-specific markers CD31, CD144, and ZO-1 localizing to cell–cell junction. QKI-7 displayed perinuclear cytoplasm localization. Scale bar: 25 μm ( c ). The expression of EC marker proteins CD31, CD144, KDR, and eNOS was shown by western blot ( d ). hiPS-ECs formed tube structure indicating their angiogenic capacity. Scale bar: 200 μm ( e ). Data are from n = 3 representative images. Source data are provided as a Source data file. Full size image The gene expression profile of one diabetic patient’s iPS-ECs, given a patient code P014, was investigated in parallel with an age-matched non-diabetic donor, donor code HD19. Compared with the non-diabetic iPS-ECs from HD19, diabetic patient iPS-ECs from P014 showed significantly higher levels of QKI-7 (Fig. 4a ), reminiscent of the miPS-ECs treated with high glucose. Consistently, the expression of CD144 , NLGN1 , and TSG6 genes and proteins was also found to be low in P014 diabetic iPS-ECs, corroborating the hyperglycemia-related dysregulation of QKI-7 and its downstream targets in turn (Fig. 4a, c, d ). Moreover, as with high-glucose-treated miPS-ECs, P014 diabetic iPS-ECs showed disrupted barrier function, decreased tube formation and increased THP-1 cell adhesion (Fig. 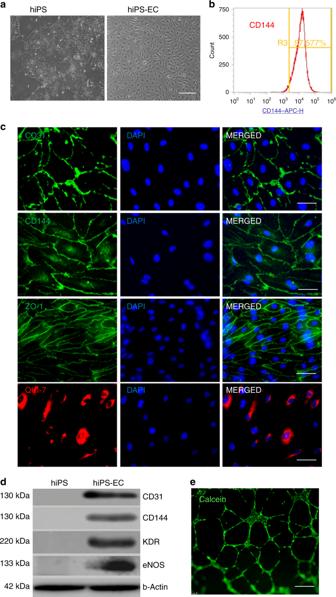4g, i, k ). Fig. 3: Human iPS cells differentiation toward ECs. Morphology of hiPSCs and their EC differentiated counterparts are shown by bright field microscopy. Scale bar: 50 μm (a). Flow cytometry showed the pure population of hiPS-derived ECs after MACS selection using CD144 magnetic beads (b). Immunofluorescence confocal image showing that the differentiated ECs expressed the EC-specific markers CD31, CD144, and ZO-1 localizing to cell–cell junction. QKI-7 displayed perinuclear cytoplasm localization. Scale bar: 25 μm (c). The expression of EC marker proteins CD31, CD144, KDR, and eNOS was shown by western blot (d). hiPS-ECs formed tube structure indicating their angiogenic capacity. Scale bar: 200 μm (e). Data are fromn= 3 representative images. Source data are provided as a Source data file. To further validate the negative regulation of the three genes by QKI-7, siRNA specifically targeting the QKI-7 isoform was transfected into iPS-ECs from P014 and the dynamics of gene expression profiles were examined. Along with efficient knockdown of QKI-7 by siRNA, CD144 , NLGN1 , and TSG6 gene/protein expression levels increased significantly, contrary to what was observed during QKI-7 overexpression in miPS-ECs (Fig. 4b, e, f ). In line with QKI-7 knockdown and the increase of functional genes in P014 diabetic iPS-ECs, major diabetic endothelial dysfunction, including increased permeability, aberrant angiogenesis, and enhanced monocyte adhesion were remarkably rescued (Fig. 4h, j, l ). With another pair of diabetic iPS-ECs, patient code P023 and age-matched non-diabetic donor HD22, a similar response to QKI-7 modification with respect to gene expression and EC functions was observed (Supplementary Fig. 6 ). Importantly, the QKI-7 high expression was detected in human coronary ECs isolated from diabetic patients (Supplementary Fig. 7A ), while QKI-7 was further increased upon high-glucose stimulation (Supplementary Fig. 7B ). Remarkably, QKI-7 expression was also detected in the blood vessels of diabetic critical limb ischemia patients (Supplementary Fig. 7C ). These findings further underline the important role of QKI-7 in the regulation of critical EC related genes, which impair EC function under diabetic conditions. Fig. 4: QKI-7 in diabetic iPS-ECs was correlated with EC dysfunction. Compared with the non-diabetic iPS-EC HD19 control, iPS-EC P014 derived from a patient with diabetes showed significantly higher level of QKI-7 ( p value: 0.0083) accompanying decreased expression of CD144, NLGN1, and TSG6 ( p values: <0.0001) ( a ). When QKI-7 was knocked down ( p value: 0.0042), iPS-ECs showed increased expression of CD144, NLGN1, and TSG6 ( p values: 0.0006, 0.0081, 0.0019) ( b ). Comparison of protein level between diabetic iPS-EC P014 and non-diabetic HD19 was shown by western blot ( c ) and ELISA ( p value: 0.0005) ( d ). Upon QKI-7 knockdown, western blot showed increase of CD144 and NLGN1 ( e ) and ELISA verified the upregulation of TSG6 ( p value: 0.0011) ( f ). Diabetic iPS-EC P014 showed significantly lower RTCA cell index than non-diabetic HD19 indicating a permeability increase ( p value: 0.0009) ( g ). When QKI-7 was knocked down, P014 RTCA cell index was enhanced, showing the alleviation of cell barrier defect ( p value: 0.0019) ( h ). Compared with the non-diabetic HD19, the diabetic iPS-EC P014 displayed more THP-1 monocyte adhesion ( p value: 0.0203) ( i ) which was ameliorated by QKI-7 knockdown ( p value: 0.0163) ( j ). In tube formation assay, diabetic iPS-EC P014 formed less capillary structure than non-diabetic HD19 cells, measured by shorter tube branch length and smaller meshed area ( p values: 0.0312, 0.0052) ( k ) which was reversed by QKI-7 knockdown ( p values: 0.0061, 0.0225) ( l ), the data were normalized by setting the control group as 1. Scale bar i , j : 100 μm; scale bar k , l : 200 μm. Data are from three biologically independent experiments. Error bars represent mean ± SEM ( n = 3). P values are shown: * p < 0.05, ** p < 0.01, *** p < 0.001, **** p < 0.0001 (two-tailed t test). Source data are provided as a Source data file. Full size image QKI-7 Binds to CD144, NLGN1 , and TSG6 promoting degradation In iPS-ECs, QKI-7 expression greatly influenced CD144 , NLGN1 , and TSG6 expression, suggesting that QKI-7 could be regulating these targets through acting as an RBP. A number of QKI-7-binding sites were predicted within the transcript sequences of the three target candidates [32] . RIP was conducted with P014 hiPS-EC lysate using QKI-7 antibody and Magna RIP kit to verify direct RNA binding by QKI-7. Using anti-QKI-7 immunoprecipitated RNA as a template, real-time RT-PCR and conventional RT-PCR validated the presence of transcripts coding for CD144 , NLGN1 , and TSG6 (Fig. 5a–d ). Fig. 5: QKI-7 promoted degradation of CD144, NLGN1, and TSG6 mRNAs. RNA immunoprecipitation (RIP) was carried out on P014 hiPS-ECs. Significantly more RNAs of CD144, TSG6, and NLGN1 were precipitated by QKI-7 antibody shown by real-time PCR and conventional PCR, indicating the direct binding of QKI-7 to transcripts of these three RNA targets ( p values: <0.0001) ( a – d ). When QKI-7 overexpressing hiPS-ECs or control cells (hiPS-ECs overexpressing an empty vector) were treated with actinomycin D in time point experiments from 0 to 12 h, the QKI-7 overexpression group showed lower mRNA level of CD144, TSG6, and NLGN1 at most of the time points as shown by the mRNA-decay curve, indicating that ectopic QKI-7 promoted mRNA degradation of the three targets ( e – g ). QKI-7 co-transfection with luciferase reporter plasmid containing wild-type 3′UTR of NLGN1 significantly suppressed the luciferase activity ( p value: 0.0329). While this effect was unobservable when QKI-7 was co-transfected with luciferase reporter plasmid containing mutated 3′UTR NLGN1 for the QKI motif ( h ). Data are from three biologically independent experiments. Error bars represent mean ± SEM ( n = 3). P values are shown: * p < 0.05, **** p < 0.0001, ns: not significant (two-tailed t test). Source data are provided as a Source data file. Full size image The cytoplasmic location of QKI-7 and its negative correlation with target mRNA levels implicate a direct impact on mRNA stability. Treatment of iPS-ECs overexpressing QKI-7 with Actinomycin D (a potent repressor of transcription), led to a decrease in transcript expression of CD144 , NLGN1 , and TSG6 at most of the time points tested compared with control cells (Fig. 5e–g ). These results evidence the pro-degradative effect of QKI-7 on target mRNAs through direct binding. Based on the RNA binding site prediction and RIP-PCR result, a QKI-7 binding motif was identified at the 3′UTR region of NLGN1 mRNA. Accordingly, a luciferase reporter construct containing a mutated QKI-7 motif in the NLGN1 3′UTR sequence was co-transfected with QKI-7 into iPS-ECs in parallel with wild-type control. Luciferase assays showed that QKI-7 combined with the wild type but not the mutant 3′UTR of NLGN1 suppressed luciferase activity, supporting the interaction of QKI-7 with the 3′UTR binding site of NLGN1 to promote mRNA degradation (Fig. 5h ). Since the QKI-7 targets NLGN1 and TSG6 are both related to vascular development, it was hypothesized that co-transfection of NLGN1 or TSG6 with QKI-7 could mitigate the anti-angiogenic impact of ectopically expressed QKI-7 . QKI-7 overexpressing iPS-ECs formed fewer capillary structure with shorter master segment length and smaller meshed area in comparison to the control cells (iPS-ECs overexpressing an empty vector) (Fig. 6a, c, d ). As expected, either NLGN1 or TSG6 co-transfection into iPS-ECs significantly alleviated the effect on tube formation caused by QKI-7 overexpression (Fig. 6b–d ). QKI-7, as an RBP, precisely regulates the expression of multiple targets linked to EC dysfunction. Indeed, both TSG6 and NLGN1 are involved in angiogenesis via regulation of EC adhesion to cell matrix. Interestingly, overexpression of either of the two genes was able to restore the disrupted EC-matrix interaction regulated by QKI-7, revealing an underlying compensatory mechanism. These findings could therefore hold great potential as a promising therapeutic target for treatment or prevention of cardiovascular complications associated with diabetes. Fig. 6: NLGN1 and TSG6 restored angiogenic capacity antagonizing QKI-7. QKI-7 overexpressing iPS-ECs formed less capillary structure with shorter master segment length ( p value: 0.0034) and smaller meshed area ( p value: 0.0016) in comparison to the control cells (iPS-ECs overexpressing an empty vector) ( a , c , d ). When NLGN1 and TSG6 were co-transfected with QKI-7 into iPS-ECs, the angiogenic capacity was recovered ( b ). No significant difference was observed between the co-transfection groups and control ( c , d ). Scale bar: 200 μm. Data are from three biologically independent experiments. Error bars represent mean ± SEM ( n = 3). P values are shown: ** p < 0.01, ns: not significant (two-tailed t test). The data were normalized by setting the control group as 1. 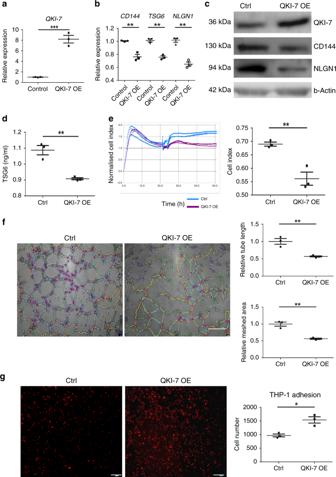Source data are provided as a Source data file. Full size image QKI-7 suppresses angiogenesis and blood flow recovery Since QKI-7 expression levels significantly impeded tube formation capacity of iPS-ECs in vitro, we next investigated the impact of QKI-7 on angiogenesis in vivo. Fig. 2: QKI-7 affected genes/proteins expression and EC functions. QKI-7 overexpression (pvalue: 0.0006) in miPS-ECs led to downregulation of EC function-related genes CD144, TSG6, and NLGN1 (pvalues: 0.0027, 0.0012, 0.0014) (a,b). Protein level alteration of QKI-7 and target candidates was verified by western blot from three independent experiments (c) and ELISA (pvalue: 0.0038) (d). QKI-7 overexpressing miPS-ECs showed decreased cell index with xCELLigence real-time cell analysis (RTCA) indicating disrupted cell barrier and increased permeability (pvalue: 0.0073) (e). In tube formation assay, QKI-7 overexpressing miPS-ECs formed less capillary structure than control cells, measured by shorter tube branch length and smaller meshed area (pvalues: 0.0069, 0.0024) (f). QKI-7 overexpression enhanced THP-1 adhesion to miPS-ECs (pvalue: 0.0107) (g), the data were normalized by setting the control group as 1. Data are from three biologically independent experiments. Error bars represent mean ± SEM (n= 3), *p< 0.05, **p< 0.01, ***p< 0.001 (two-tailedttest). The source data are provided as a Source data file. iPS-ECs overexpressing QKI-7 in parallel with control cells (iPS-ECs overexpressing an empty vector) were mixed with Matrigel and injected subcutaneously into C57BL/6 mice for 7 days. Immunohistochemistry of the harvested Matrigel plugs demonstrated that the QKI-7 overexpressing iPS-ECs formed fewer capillary structures with irregular organization compared with the control cells, corroborating the angiogenic deficiency of iPS-ECs due to QKI-7 upregulation (Fig. 7a ). In contrast to the control cells group, QKI-7 overexpression group also showed an interrupted angiogenetic capacity of ECs demonstrated by hematoxylin and eosin staining and quantification (Supplementary Fig. 8A–C ). Furthermore, the impact of QKI-7 expression on arteriogenesis under diabetic condition was tested in vivo. The murine hindlimb ischemia model is a well-established strategy for in vivo assessment of arteriogenesis [33] . The occurrence of limb ischemia is highly correlated with diabetes and diabetes patients with coronary artery disease, who have fewer collateral vessels compared with patients without diabetes [34] . In this study, intramuscular injection of either QKI-7 -expressing miPS-ECs or control cells (iPS-ECs overexpressing an empty vector) was performed immediately after induction of hindlimb ischemia in STZ-induced diabetic mice. PBS was also used as an additional control. After 14 days, delivery of control miPS-ECs significantly promoted the blood flow recovery of the ischemic hindlimb, as indicated by Laser Doppler imaging, however, the angiogenesis-enhancing effect of miPS-EC transplantation was substantially compromised in the QKI-7 overexpression group (Fig. 7b ). Fig. 7: QKI-7 affected blood reperfusion of the ischemic hindlimbs. Matrigel plug assay was carried out using QKI-7 overexpressing miPS-ECs or control cells. In contrast to the control group, QKI-7 overexpression group formed much fewer capillary structures ( p value: 0.0096) with irregular organization, suggesting an interrupted angiogenetic capacity of ECs ( a images and quantification from 9 plugs per group based on n = 3 biological replicates). Hindlimb ischemia was induced in STZ-diabetic mice and QKI-7 overexpressing or control miPS-ECs were injected into the adductors immediately after induction of hind limb ischemia. Laser Doppler images of blood flow in the lower limbs of mice in prone position, with the ischemic leg highlighted by the yellow rectangle. After 14 days, delivery of control miPS-ECs significantly promoted the blood flow recovery of the ischemic hind limb, which was substantially compromised in the QKI-7 overexpression group ( p values: 0.0018, 0.0037) ( b ). In vivo QKI-7 knockdown was achieved by intramuscular injection of shRNA Lentivirus construct tagged with a CD144 promoter and GFP to target ECs, and blood flow recovery in STZ-diabetic mice was investigated. The QKI-7 knockdown group showed over 60% of perfusion ratio to the opposite intact limb which was significantly higher than the scrambled Lentivirus control group ( p value: 0.0081) ( c ). The effects of blood flow recovery in the QKI-7 knockdown group were also confirmed by hematoxylin and eosin staining where increased capillary density is shown ( p value: 0.0062) ( d ). The downregulation of QKI-7 by shRNA lentivirus was verified by immunohistochemistry, when the adductor tissue was harvested, fixed, cryosectioned, and stained. Compared with the scrambled control, the QKI-7 knockdown group showed significantly higher expression of EC marker CD144 along with QKI-7 suppression ( p values: 0.0072, 0.0056) ( e ). GFP staining clearly shown that the Lentiviral constructs tagged with GFP targeted ECs in vivo ( e ). Scale bar: a 200 μm; d 100 μm; e 200 μm. Data are from three biologically independent experiments. Error bars represent mean ± SEM ( n = 3). P values are shown: ** p < 0.01, ns: not significant (two-tailed t test). Source data are provided as a Source data file. Full size image Targeting QKI-7 in vivo restores EC function in diabetic mice The effect of QKI-7 knockdown on the reperfusion of hindlimb ischemia in diabetic mice was next examined by shRNA Lentivirus infection. A QKI-7 shRNA Lentivirus construct containing the CD144 promoter and tagged with GFP enabled direct targeting of ECs in vivo and was injected intramuscularly immediately after induction of hindlimb ischemia in STZ-induced diabetic mice. A non-targeting (NT) shRNA Lentivirus construct containing the CD144 promoter and tagged with GFP, and PBS were used as additional controls. Compared with the NT lentivirus control, QKI-7 knockdown significantly promoted blood flow recovery of the ischemic hindlimb in diabetic mice (Fig. 7c ). These findings were also confirmed by performing hematoxylin and eosin staining where increased capillary density is shown in Fig. 7d (images and quantification). Importantly, the perfusion ratio of the QKI-7 shRNA lentivirus treatment group reached ~60%, which was around double that observed in the scrambled control-injected diabetic mice. The efficient downregulation of QKI-7 by shRNA lentivirus was verified by immunohistochemistry in the adductor tissue harvested (Fig. 7e ). Since the lentiviral constructs were tagged with GFP, the specificity of targeting ECs is shown in Fig. 7e , where GFP staining was detected in cells co-expressing the EC marker CD144. Notably, higher levels of CD144 accompanied with a decrease in QKI-7 was observed, consistent with the upregulation of CD144 by QKI-7 knockdown in mouse and human iPS-ECs (Fig. 7e , and quantification). Moreover, HRP-DAB immunohistochemical staining with CD31 on the sections injected with lentiviral shQKI-7 (KD), confirmed the above findings, and further shown increased arterioles and venule density (Supplementary Fig. 9A–C , and quantification in D). HRP-DAB immunohistochemical staining for the smooth muscle marker SMA is also shown in (Supplementary Fig. 9E, F ). In parallel, the efficiency of the shQKI-7 construct (pLV[miR30-shRNA]-Cd144>EGFP) was also tested in vitro when iPS-ECs were infected by lentiviral gene transfer and the cells were harvested 72 h later, and the expression levels of QKI-7 were tested (Supplementary Fig. 10 ). These data validated the important role of QKI-7 in driving angiogenesis/arteriogenesis and neovascularisation in diabetes, restoring EC function. Furthermore, these findings indicate the clinical implication of reducing the expression of QKI-7 may be a potential therapeutic strategy for the treatment of diabetic complications. In this study, the expression of QKI-7 in diabetic human iPS-ECs was found to be high in line with its increased levels observed in high-glucose-treated miPS-ECs. In addition, QKI-7 was found to be highly expressed in human coronary arterial ECs isolated from diabetic donors, and in blood vessels isolated from diabetic critical limb ischemia patients, QKI-7 expression was also detected. Overexpression of QKI-7 in iPS-ECs demonstrated impaired barrier function and compromised tube formation capability as well as increased monocyte adhesion, which are hallmark features of endothelial dysfunction in diabetes. These results were also verified in diabetic iPS-ECs when compared with non-diabetic donors; the functional defects observed in diabetic iPS-ECs were partly rescued with QKI-7 knockdown, strongly supporting our conclusion that QKI-7 contributes to the pathogenesis of diabetic EC dysfunction. Of note, the expression levels of the other isoforms, QKI-5 and QKI-6 , were not affected in either diabetic iPS-ECs or high-glucose-treated miPS-ECs, suggesting that a specific alternative splicing mechanism is associated with QKI-7 isoform transcript generation under diabetic conditions. By screening possible splicing factors that bind to QKI-7 , CUG-BP , and hnRNPM were found to be involved. Interestingly, the two candidates showed diametrically opposed dynamics, with high glucose upregulating CUG-BP while decreasing hnRNPM . In addition, the level of QKI-7 was upregulated and downregulated by CUG-BP and hnRNPM overexpression, respectively, while direct binding to QKI-7 was demonstrated by RIP assays. Therefore, it appears that CUG-BP and hnRNPM may diametrically regulate QKI-7 expression at the post-transcriptional level to maintain homeostasis. This balance was further abrogated by the observed CUG-BP increase and hnRNPM reduction under hyperglycemic conditions, leading to upregulation of QKI-7 . hnRNPs are RBPs that play crucial roles in pre-mRNAs processing, mRNA decay, and translational regulation. hnRNPM has been well studied in the transcription regulation of genes related to epithelial–mesenchymal transition (EMT), and TGFβ signaling [35] . Collectively, hnRNPM competitively binds to G/U rich motifs and regulates genes related to cell adhesion, migration, and cytoskeleton organization [36] . CUG-BP is a multifunctional RBP that regulates pre-mRNA alternative splicing, mRNA stability, mRNA editing, and translation [37] . CUG-BP is highly expressed in the pancreatic islets of diabetic mice [38] . In diabetic cardiomyopathy, CUG-BP overexpression was also observed and contributed to cardiac complications [39] . CUG-BP was found to bind to the 3′ UTRs and negatively regulate the half-lives of transcripts encoding the RBPs CELF2 , Mbnl1 , and Mbnl2 [40] , [41] . With this in mind, these previous reports and our current finding of QKI-7 as another CUG-BP target, it seems likely that CUG-BP acts as an important upstream factor regulating the transcription network in diabetes. Along these lines, targeting CUG-BP could therefore provide a potential strategy to treat diabetic complications. Using the defined QRE bipartite consensus sequence NACUAAY-N1–20-UAAY 1430 mRNA target candidates of QKI proteins were identified [25] . From this published database, we selected 35 putative QKI target genes for exploration of QKI-7’s downstream effectors based on their relevance to vascular EC functions. With QKI-7 overexpression, the expression of CD144 , NLGN1 , and TSG6 was downregulated, while their expression was increased with QKI-7 knockdown. Furthermore, RIP assays and mRNA stability assays verified that QKI-7 destabilized their mRNA through direct target binding. In our previous work, QKI-5 was reported to induce increased CD144 levels in iPS-ECs by stabilizing CD144 mRNA [22] , which is contrary to the current finding with QKI-7 . All QKI family isoforms share the same KH RNA-binding domain and only differ at the C-terminus. Thus, QKI-5 and QKI-7 might compete for binding to CD144 mRNA and recruit different post-transcriptional machinery to impact mRNA turnover in an antagonistic manner. CD144 is a critical component of EC adherens junctions that regulates barrier integrity and angiogenesis [26] , [42] . Due to enhanced QKI-7 binding and mRNA degradation, CD144 reduction under hyperglycemic conditions may therefore contribute to defective EC barrier function as well as compromised angiogenesis. TSG6 is a TNFα/IL-1-inducible secretory protein and contains a hyaluronan-binding domain homologous to the N122-terminal half of CD44 and participates in the regulation of cell–cell interactions [27] . Disruption of the functional interaction between TSG6 and hyaluronan with a specific antibody severely altered ECM formation [43] . TSG6 has also been shown to be a potent anti-inflammatory factor. On the other hand, when TSG6 was knocked down, the anti-inflammatory effects of human mesenchymal stromal cells were abolished [28] , [44] . One of the underlying mechanisms is interaction of TSG6 with CD44 to suppress NF-kB signaling [45] , [46] , [47] . In diabetic mice, subconjunctival injections of recombinant TSG6 promoted corneal epithelial wound healing through activation of resident progenitor cells and acceleration of M2 macrophage polarization [48] . Atherosclerosis is one of the major diabetic complications and inflammatory events in the vascular endothelium. When harmed by oxidative stress and other factors associated with diabetes, activated ECs release cytokines and chemokines to attract monocytes that adhere and develop into macrophages and foam cells, ultimately driving atherogenesis [49] , [50] . The current study revealed that QKI-7 controlled downregulation of TSG6 in diabetic ECs, and that THP-1 monocyte adhesion was decreased after QKI-7 knockdown and TSG6 expression level restoration, suggesting that as a potent anti-inflammatory factor, TSG6 maintains vascular EC function and inhibits atherogenesis. NLGN1 is a cell surface protein that was originally found to be involved in synaptic transmission through cell–cell interaction and collaboration with neurexin family members. Recently, NLGN1 was reported to play an important role in vascular development [51] , [52] , [53] . In vitro, NLGN1 demonstrated abundant expression in vascular ECs and NLGN1 expression dynamics significantly affected the tube formation capacity of ECs. In vivo, NLGN1 knockout caused structural defects in the vascular tree of the developing mouse retina with disrupted cell–cell junctions and aberrant distribution of laminin, VE-cadherin and α6 integrin. Our present study is in agreement with the above reports that NLGN1 is correlated with the tube formation capacity of ECs. Further to the observed negative regulation of QKI-7, NLGN1 downregulation in ECs may therefore play an important role in the ontology of diabetic EC dysfunction. Defective angiogenesis associated with vascular endothelial dysfunction is a shared abnormality in many diabetic complications, including ischemic cardiovascular disease and wound healing deficiencies. Failure to respond to ischemia by promoting angiogenesis is intimately correlated with poor clinical outcomes in diabetes. In STZ-induced diabetic mice, the recovery of blood flow was significantly compromised after ligation or excision of the common femoral artery with the ischemic hindlimb showing fewer collateral arteries visible on angiography [54] , [55] . Our current study presents a similar result further to evaluation of hindlimb hemodynamics following induction of ischemia in diabetic mice. Interestingly, when QKI-7 was knocked down by shRNA lentivirus infection targeting endogenous ECs in diabetic mice in vivo, blood flow recovery in ischemic hindlimbs was dramatically improved. 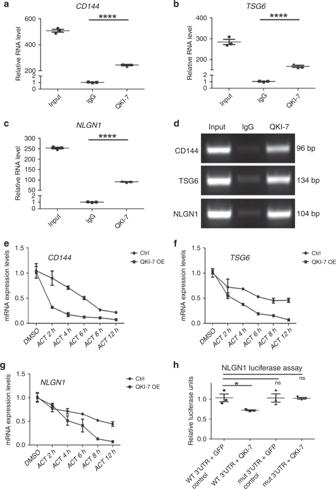Fig. 5: QKI-7 promoted degradation of CD144, NLGN1, and TSG6 mRNAs. RNA immunoprecipitation (RIP) was carried out on P014 hiPS-ECs. Significantly more RNAs of CD144, TSG6, and NLGN1 were precipitated by QKI-7 antibody shown by real-time PCR and conventional PCR, indicating the direct binding of QKI-7 to transcripts of these three RNA targets (pvalues: <0.0001) (a–d). When QKI-7 overexpressing hiPS-ECs or control cells (hiPS-ECs overexpressing an empty vector) were treated with actinomycin D in time point experiments from 0 to 12 h, the QKI-7 overexpression group showed lower mRNA level of CD144, TSG6, and NLGN1 at most of the time points as shown by the mRNA-decay curve, indicating that ectopic QKI-7 promoted mRNA degradation of the three targets (e–g). QKI-7 co-transfection with luciferase reporter plasmid containing wild-type 3′UTR of NLGN1 significantly suppressed the luciferase activity (pvalue: 0.0329). While this effect was unobservable when QKI-7 was co-transfected with luciferase reporter plasmid containing mutated 3′UTR NLGN1 for the QKI motif (h). Data are from three biologically independent experiments. Error bars represent mean ± SEM (n= 3).Pvalues are shown: *p< 0.05, ****p< 0.0001, ns: not significant (two-tailedttest). Source data are provided as a Source data file. On the other hand, QKI-7 overexpression in iPS-ECs substantially inhibited their pro-angiogenic effect when transplanted in diabetic mice, indicating that QKI-7 serves an effective anti-angiogenic function. Of the three QKI-7 targets discovered in the current study, CD144 is a well-known endothelial adhesion molecule that is critical for intercellular junction and vascular development. Likewise, both TSG6 and NLGN1 participate in regulation of EC-cell–matrix interaction which is critical for vasculogenesis. Downregulation of these important angiogenesis-related factors by QKI-7 therefore partly explains its negative impact on angiogenesis. While diabetic endothelial dysfunction-related angiogenesis deficiency is multifactorial, and a number of therapeutic regimens have been investigated for the treatment of chronic ischemic disorders and diabetic wound healing, current clinical strategies are incompletely effective due to the limited specific therapeutic targets of these methodologies [56] . In our study, in vitro rescue assay verified that reduced QKI-7 expression ameliorated diabetic EC dysfunction, namely defective barrier formation, impaired angiogenesis, and increased adhesion of monocytes. In addition, in vivo downregulation of QKI-7 in diabetic mice exerted positive effects on angiogenesis, promoting the blood flow recovery of ischemic hindlimbs. Taken together, these findings suggest that QKI-7 may represent a potential target for the treatment of diabetic complications. Importantly, as an upstream RBP, QKI-7 has potential to work as a key negative regulator to modulate multiple effectors and to impact various aspects of EC function, including barrier integrity, angiogenesis and inflammation. Therefore, specific modulation of QKI-7 levels is likely to be superior to therapeutic strategies directed toward individual targets to reduce diabetic complications. There are still some questions that need to be answered in relation to the functional features and underlying mechanisms of QKI-7 signaling. First, there are multiple mRNA transcripts containing the defined QRE bipartite consensus sequence [25] , so it is conceivable that there are more RNA-binding targets for QKI-7 under diabetic conditions. Our ongoing RIP-seq work is aimed at exploring more QKI-7 binding targets so that a more comprehensive, QKI-7-centered regulation network may be built to better understand the underlying mechanisms and identify powerful targets for diabetes treatment. Second, specific signaling pathways involved in the dysregulation of CUG-BP/hnRNPM/QKI-7 in diabetes need to be elucidated. For example, aberrant PKC signaling activation has been investigated in diabetic cardiomyopathy [57] and activated PKC isozymes α/β were revealed to contribute to abnormal alternative splicing through phosphorylation and upregulation of CUG-BP/Rbfox2 proteins. Third, it is important to define how QKI isoforms are able to work distinctly via specific C-termini. The C-terminal region of QKI-7 (-EWIEMPVMPDISAH-) contains three negatively charged residues and theoretical pI of 4.13 ( https://web.expasy.org/protparam/ ), which is quite different from that of QKI-5 (-GAVATKVRRH DMRVHPYQRI VTADRAATGN-), which contains 6 positively charged residues with theoretical pI of 11.44, and that of QKI-6 (-GMAFPTKG-), with theoretical pI of 8.75. The distinctive C-terminal composition of QKI isoforms thereby determines their difference in partner recruitment, complex formation, and influences on stability of RNA targets and functions. A possible strategy would be to design small molecules against the QKI-7 C-terminus, based on crystallographic structure elucidation, to promote development of specific and effective clinical applications. In summary, the present study provides key insight into the important role of QKI-7 in the pathogenesis of EC dysfunction associated with diabetes. Imbalance of CUG-BP/hnRNPM regulation in diabetic ECs leads to upregulation of QKI-7, which in turn enhances mRNA degradation of RNA-binding targets, CD144, TSG6, and NLGN1. This subsequently contributes to diabetic endothelial dysfunction, including increased permeability, impaired tube formation and increased monocyte adhesion (as summarized in Supplementary Fig. 11 ). Such results indicate that QKI-7 is at least partly responsible for vascular complications in diabetes making it an attractive target for developing therapeutic diabetes treatment strategies. Mouse and human iPSC culture and differentiation Mouse iPSCs were generated in our laboratory by transfection of pCAG2LMKOSimO vector expressing c-Myc, Klf4, Oct4, and Sox2 into MEFs [58] , [59] , and cultured in gelatin-coated flasks (PBS; Life Technologies 10010056 containing 0.02% gelatin from bovine skin; Sigma-Aldrich G1393) in DMEM (ATCC 30-2002) supplemented with 10% fetal bovine serum (FBS) (Embryomax; Millipore ES-009-B), 100 IU/ml penicillin, and 100 μg/ml streptomycin (PenStrep) (Thermo Fisher Scientific 10378-016), 10 ng/ml recombinant human leukemia inhibitory factor (Millipore LIF1010) and 0.1 mM 2-mercaptoethanol (Life Technologies 31350-010) in a humidified incubator supplemented with 5% CO 2 . Cells were passaged every 2 days at a ratio of 1:6. EC differentiation of iPSCs was induced by seeding the cells on type IV mouse collagen (5 μg/ml; R&D Systems 3410-010-01)-coated dishes in differentiation medium (DM) containing α-MEM (Life Technologies 32571036) supplemented with 10% FBS (Invitrogen 10270106), 0.05 mM 2-mercaptoethanol, 100 units/ml penicillin, and 100 μg/ml streptomycin in the presence of 25 ng/ml VEGF (Thermo Fisher Scientific PMG0111) for the time points indicated. For high-glucose treatment, culture medium was supplemented with D-glucose to reach concentrations indicated in the Figures. L-glucose was used as controls in these experiments. Diabetic patient-specific iPSCs were generated based on a protocol which we have recently reported [30] . Mononuclear cells from donor peripheral blood were expanded and reprogrammed into iPS cells by transfection of nonintegrating episomal plasmid vectors pEB-C5 (overexpressing Oct4, Sox2, Klf4, c-Myc, and Lin28), and pEB-Tg vector (overexpressing SV40 large T antigen). The pluripotency and germ layer differentiation capacity of the generated iPS lines were verified. Ethical approval was obtained from the Office for Research Ethics Committees of Northern Ireland (ORECNI) (REC 14/NI/1109). Verbal and written information about the study was provided to all participants and written informed consent was obtained prior to study procedures from those willing and consenting to take part. Patients with type 1 and type 2 diabetes of more than 15 year standing and age- and sex-matched non-diabetic volunteers, who acted as controls, were recruited to this study. Patients unable to provide informed consent for the study were excluded. All the iPS cells-based in vitro and in vivo studies were confirmed in two independent non-diabetic and two diabetic donors sets based on three biological replicates with n = 3. The QKI-7 expression was also verified in four additional iPS-ECs lines generated from four independent (sex and age-matched) diabetic donors, based on three biological replicates with n = 3. On the day of blood sample collection, a detailed medical history was obtained and blood pressure was measured. A 20 ml sample of peripheral blood was obtained by venepuncture into VACUETTE® K3 EDTA-coated 4-ml tubes (454021, GREINER Bio-One). Human iPSCs were cultured using mTeSR-1 medium (Stemcell 85850) following the manufacturer’s instructions. For EC differentiation, iPSCs were first cultured for 3 days in a 1:1 mixture of DMEM/F-12 (Thermo Fisher Scientific 31330038) with Neurobasal medium (Thermo Fisher Scientific 21103049) supplemented with N2 (Thermo Fisher Scientific 17502048), B27 (Thermo Fisher Scientific 17504044), 8 µM CHIR99021 (Sigma-Aldrich SML1046), and 25 ng/ml BMP4 (Life Technologies PHC9534). Thereafter, the cells were cultured for 2 days in StemPro 34 medium (Thermo Fisher Scientific 10639011) supplemented with 200 ng/ml hVEGF (Life Technologies PHC9391) and 2 µM Forskolin (Sigma-Aldrich F6886). On day 6, CD144 positive cells were magnetically sorted using MicroBeads Kit (Miltenyi BIotec 130-097-857) and cultured in EGM-2 media (LONZA 00190860). Human coronary artery endothelial cells were purchased from Lonza: HCAEC Coronary Art Endo Cells (CC-2585), DHCAEC Human Coronary Art Endo Cells Diabetic (CC-2921). The cells were cultured in EGM-2 media (LONZA 00190860). All methods regarding the mouse and human iPSC culture and differentiation were performed in accordance with the relevant institutional guidelines and regulations including Declaration of Helsinki and Ethical Guidelines for Medical and Health Research Involving Human Subjects. Glucose treatment in human fibroblasts L-Glucose (G5500) or D-glucose (G7021), both from Sigma, were reconstituted in fibroblast media (10% FBS F-12K medium (Kaighn’s modification of Ham’s F-12 medium) by ATCC (30-200). Fibroblasts (HFL1 (ATCC® CCL-153™)) were seeded in 6-well plates in 2 ml media per well at a seeding density of 100,000 or 200,000 cells for a total of 6 and 3 days of glucose treatment, respectively. Cell culture media were substituted on day 2 and on day 4. After the initial glucose treatment on day 0, the treatments were repeated with L- or D-glucose at a final concentration of 30 mM on day 2 and day 4 until harvested for subsequent real-time PCR analysis. RNA silencing The SiRNA duplex for specific silencing of QKI-7 was synthesized (Sigma-Aldrich). The SiRNA sequence was -GUGAGGAGAUUGGUAUUAGUU-. A total of 1 × 10 6 iPS-ECs were resuspended in Nucleofector® solution, mixed with 5-µM SiRNA and transferred into an amaxa certified cuvette. A scrambled SiRNA (Thermo Fisher AM4611) was used as control. After 48 h, the cells were harvested for quantification of gene and protein levels of QKI-7 . Constructs for gene manipulation and luciferase assays QKI-7 ORF was cloned into pReceiver-Lv225 vector to generate QKI-7 overexpression construct (GeneCopoeia). For lentivirus packaging, 1 × 10 7 293-T cells were transfected with QKI-7 overexpression plasmid, pCMV-dR8.2 (Addgene 8455), pCMV-VSV-G (Addgene 8454), and Endofectin (GeneCopoeia EFM1004). The supernatant containing the lentivirus was harvested twice at 48 and 96 h later, filtered (0.45 µm) and stored at −80 °C. Overexpression constructs for hnRNPM (plasmid #64924), CUG-BP (plasmid #61276) and NLGN1 (plasmid #15260) were obtained from Addgene. TSG6 (NM_007115.3) ORF was cloned into the 3rd generation of lentivirus vector to generate TSG6 overexpression construct (VectorBuilder). 3′ UTR sequence of NLGN1 was obtained by RT-PCR and cloned downstream of luciferase (hLuc) reporter gene in a Firefly/Renilla Duo-Luciferase reporter vector pEZX-MT06 (GeneCopoeia). Plasmid transfections were performed using Endofectin following the manufacturer’s instructions. Quantitative real-time polymerase chain reaction (RT-PCR) Total RNA was extracted using the RNeasy Mini Kit (Qiagen 74104) according to the manufacturer’s protocol. 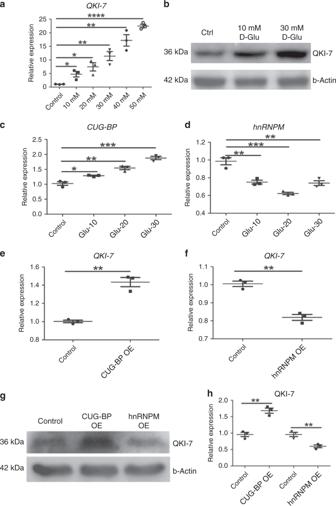Two micrograms of RNA were reverse transcribed into cDNA with random primer by reverse transcriptase (RT) (Thermo Fisher Scientific 4374966). Relative gene expression was determined by quantitative real-time RT-PCR, using 20 ng cDNA (relative to RNA amount) for each sample with the SYBR Green Master Mix (Thermo Fisher Scientific A25742) in a 10 μl reaction. Ct values were measured using a LightCycler 480 sequence detector (Roche). GAPDH served as the endogenous control to normalize the amounts of RNA in each sample. Fig. 1: QKI-7 dynamics under high glucose related to CUG-BP and hnRNPM. Upon high-glucose treatment of miPS-ECs, QKI-7 expression showed a dose-dependent increase at both mRNA (pvalues: 0.023, 0.013, 0.0034, 0.0016, and <0.0001) and protein levels (a,b). CUG-BP was upregulated by high-glucose treatment dose-dependently (pvalues: 0.013, 0.0032, 0.0004) (c). hnRNPM expression was downregulated by high-glucose treatment (pvalues: 0.0064, 0.001, 0.0069) (d). CUG-BP overexpression enhanced QKI-7 expression (pvalue: 0.0012) (e). hnRNPM overexpression suppressed QKI-7 expression (pvalue: 0.0011) (f). QKI-7 upregulation by overexpressed CUG-BP and downregulation by ectopic hnRNPM is shown by western blot (g) and quantified in (h) (pvalues: 0.0021, 0.0099). L-glucose-treated cells have been used as controls in these experiments. Data are from three biologically independent experiments. Error bars represent mean ± SEM (n= 3).Pvalues are shown: *p< 0.05, **p< 0.01, ***p< 0.001, ****p< 0.0001 (two-tailedttest). The source data are provided as a Source data file. The primers are shown in Supplementary Table 1 . Enzyme-linked immunosorbent assay The concentration of TSG6 released into the supernatant of 6-day differentiated ECs was detected by TSG6 ELISA (Sigma-Aldrich RAB1092) according to the manufacturer’s procedure. Western blot Cells were harvested and washed with cold PBS, resuspended in lysis buffer (25 mM Tris-Cl pH 7.5, 120 mM NaCl, 1 mM EDTA pH 8.0, 0.5% Triton X-100) supplemented with protease inhibitors (Roche 11697498001) and lysed by ultra-sonication (twice, for 6 s) (Bradson Sonifier150) to obtain whole-cell lysate. The protein concentration was determined using the Bradford Dye Reagent (Bio-Rad 500-0205). Fifty micrograms of whole lysate was applied to SDS-PAGE and transferred to Hybond PVDF membrane (GE Health 15259894), followed by standard western blot procedure. Flow cytometric analysis iPSCs derived ECs were dissociated by incubation with 0.05% Trypsin-EDTA (Thermo Fisher Scientific 25300054) for 5 min at 37 °C. A total of 1 × 10 6 single cells were resuspended in 100 μl FACS buffer (PBS supplemented with 10% FBS) and stained by incubation with 5 μl CD144-APC antibody for 30 min at 4 °C in the dark. The cells were washed twice with PBS before resuspension in 1 ml PBS for FACS experiment on an Attune NxT Flow Cytometer and data were analyzed with Attune software (Thermo Fisher Scientific). Antibodies The bound primary antibodies were detected by the use of horseradish peroxidase (HRP)-conjugated secondary antibodies by Bio-Rad (170-6515, 170-6516, 1:3000) and the ECL detection system (GE Health GERPN2232). Primary antibodies include QKI-7 (UC Davis/NIH NeuroMab Facility 73-200, WB 1:1000, ICC 1:100), CD144 (St John’s Laboratory STJ96234, WB 1:1000, ICC 1:200), CD31 (Abcam AB28364, WB 1:1000, ICC 1:20), KDR (R&D Systems MAB3571, WB 1:1000), FLK1 (Thermo Fisher Scientific MA5-15157, WB 1:1000), eNOS (Abcam AB76198, WB 1:1000), NLGN1 (Abcam ab153821, WB 1:1000), β-actin (R&D Systems MAB8928, WB 1:1000), and ZO-1 (Thermo Fisher Scientific 40-2200, ICC 1:200). For immunofluorescence staining, Alexa Fluor secondary antibodies were used (Thermo Fisher Scientific A21202, A11057, A28175, A11004, A11055, A11008, 1:500). For flow cytometry, CD144-APC (Thermo Fisher Scientific 17-1449-42, 1:20) and Mouse IgG1 kappa Isotype Control-APC (Thermo Fisher Scientific 17-4714-82, 1:800) were used. Luciferase reporter assay For luciferase reporter assays, 4 × 10 4 /well of iPS-ECs were seeded on collagen-coated wells of a 12-well plate in EGM-2 medium. 0.33 μg/well of reporter plasmids were co-transfected with QKI-7 or control (0.17 μg/well) plasmids using Endofectin Transfection Reagent (GeneCopoeia EFM1004) according to the protocol provided. pGL3-Luc Renilla (0.1 μg/well) was included in all transfection assays as an internal control. Luciferase and Renilla activity assays were detected 48 h after transfection using Dual-Glo Luciferase Assay System (Promega E2920). Relative luciferase units (RLU) was defined as the ratio of luciferase activity to Renilla activity with that of control set as 1. RNA-binding protein (RBP) immunoprecipitation assays RBP immunoprecipitation assays were performed on iPS-ECs using the Magna RIP kit from Millipore (17-700) according to the protocol provided. A QKI-7 specific antibody from Millipore, CUG-BP (PA5-85997), hnRNPM (MA1-91607) and mouse or rabbit IgG-purified antibodies were used. The precipitated RNA was subjected to RT-PCR using specific primers for the binding sites of QKI , CUG-BP , and hnRNPM motifs. Immunofluorescence cell staining Cells were fixed with 4% paraformaldehyde and permeabilized with 0.1% Triton X-100 in PBS for 10 min and blocked in 5% swine or donkey serum in PBS for 30 min before incubation with primary antibodies, previously mentioned, for 1 h at 37 °C. Alexa Fluor secondary antibodies by Thermo Fisher Scientific were incubated for 45 min at 37 °C. Cells were counterstained with 4′,6-diamidino-2-phenylindole (DAPI; Sigma-Aldrich), mounted in Fluoromount-G (Cytomation; DAKO, Glostrup, Denmark), and imaged using a fluorescent (Axioplan 2 imaging; Zeiss) or confocal microscope (SP5, Leica, Germany). Immunofluorescence tissue staining Tissues were fixed with cold acetone (4 °C), washed with TBS and blocked in 5% donkey serum in TBS for 2 h at room temperature in a humidified atmosphere before incubating with primary antibodies overnight at 4 °C. The following day, Alexa Fluor secondary antibodies were incubated for 45 min at 37 °C and DAPI solution (62248, Thermo Fischer Scientific) for 5 min at room temperature. Tissues were mounted on VectaShield Antifade Mounting Medium (H-1000) and imaged using a fluorescent (80i Eclipse; Nikon, Japan) or confocal microscope (SP8, Leica, Germany). Hematoxylin and eosin staining Tissue sections were rinsed in tap water for 5 min to hydrate and then stained with Harris’ hematoxylin solution (Leica 381560E) for 5 min at room temperature. Tissues were then rinsed in tap water for 3 min. Next, tissues were dipped in 1% acid ethanol (1% HCL + 70% alcohol aq. Leica 3801590E) for 10 s and then soaked into 1% ammonia in H 2 O for 30 s. Tissues were then placed into filtered eosin solution (Leica 3801590E) for 3 min. Tissues were next dehydrated with 75, 95, and 100% absolute ethanol. Finally, for the clearing step, tissues were rinsed with clearing agent (Leica 3803600E) for 9 min and slides were mount with DPX mountant (Sigma 06522). IHC staining Sections were air-dried at RT for 15–20 min. Sections were next rinsed shortly with tap water and incubated for 10 min in cold 1:1 acetone:methanol solution and let them dry for 40 min at RT. Sections were then permeabilized with 0.2% Triton X-100 in TBS for 10 min at RT. And washed with 0.025% TBS-T for another 15 min. Next sections were blocked with BLOXALL® Blocking Solution (30150 ZF0726) for 10 min at RT (Peroxidase blocking) and washed with 0.025% TBS-T for another 15 min at RT. Sections were then blocked for 2 h at room temperature with 5% Donkey serum in 1% BSA in 0.025% TBS-T, and incubated overnight at 4 °C with primary antibody (aSMA Ab5694 and CD31 Ab28364). Next day, sections were washed with 2 × 5 min with TBS and blocked in 0.3% H 2 O 2 in TBS for 15 min at RT. Tissues were then incubated with secondary antibody (goat anti-rabbit, Bio-Rad, Cat. 1706515) in 5% donkey serum, 1% BSA, and in 0.025% TBS-T for 45 min at 37 °C in humidity DAB solution (K4010, lot 015095) and Dab Substrate buffer (K4006 Lot 104224) was then applied to tissue sections for 10 min in the dark, and washed for 15 min with 0.025% TBS-T and for another 5 min rinsed with tap water. Finally, tissues were stained with haematoxylin blue as described in our H&E staining omitting the eosin incubation step. In vitro tube formation assay Hundred microliters of Matrigel (Corning 356231) was distributed into wells of a 96-well plate using pre-cooled tips and incubated at 37 °C for 1 h. A total of 1 × 10 4 iPS-ECs were seeded onto the Matrigel bed of each well and incubated at 37 °C. 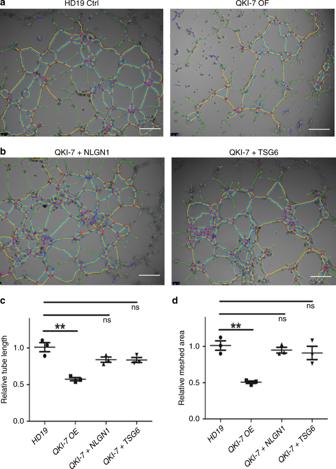Fig. 6: NLGN1 and TSG6 restored angiogenic capacity antagonizing QKI-7. QKI-7 overexpressing iPS-ECs formed less capillary structure with shorter master segment length (pvalue: 0.0034) and smaller meshed area (pvalue: 0.0016) in comparison to the control cells (iPS-ECs overexpressing an empty vector) (a,c,d). When NLGN1 and TSG6 were co-transfected with QKI-7 into iPS-ECs, the angiogenic capacity was recovered (b). No significant difference was observed between the co-transfection groups and control (c,d). Scale bar: 200 μm. Data are from three biologically independent experiments. Error bars represent mean ± SEM (n= 3).Pvalues are shown: **p< 0.01, ns: not significant (two-tailedttest). The data were normalized by setting the control group as 1. Source data are provided as a Source data file. 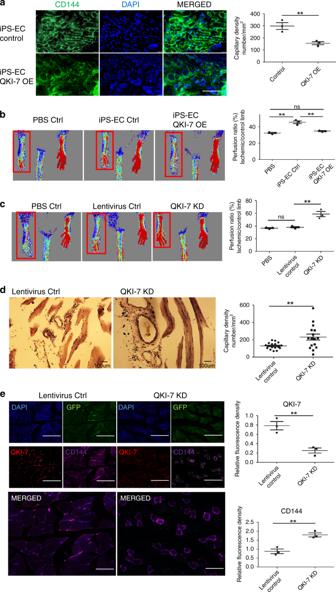Fig. 7: QKI-7 affected blood reperfusion of the ischemic hindlimbs. Matrigel plug assay was carried out using QKI-7 overexpressing miPS-ECs or control cells. In contrast to the control group, QKI-7 overexpression group formed much fewer capillary structures (pvalue: 0.0096) with irregular organization, suggesting an interrupted angiogenetic capacity of ECs (aimages and quantification from 9 plugs per group based onn= 3 biological replicates). Hindlimb ischemia was induced in STZ-diabetic mice and QKI-7 overexpressing or control miPS-ECs were injected into the adductors immediately after induction of hind limb ischemia. Laser Doppler images of blood flow in the lower limbs of mice in prone position, with the ischemic leg highlighted by the yellow rectangle. After 14 days, delivery of control miPS-ECs significantly promoted the blood flow recovery of the ischemic hind limb, which was substantially compromised in the QKI-7 overexpression group (pvalues: 0.0018, 0.0037) (b). In vivo QKI-7 knockdown was achieved by intramuscular injection of shRNA Lentivirus construct tagged with a CD144 promoter and GFP to target ECs, and blood flow recovery in STZ-diabetic mice was investigated. The QKI-7 knockdown group showed over 60% of perfusion ratio to the opposite intact limb which was significantly higher than the scrambled Lentivirus control group (pvalue: 0.0081) (c). The effects of blood flow recovery in the QKI-7 knockdown group were also confirmed by hematoxylin and eosin staining where increased capillary density is shown (pvalue: 0.0062) (d). The downregulation of QKI-7 by shRNA lentivirus was verified by immunohistochemistry, when the adductor tissue was harvested, fixed, cryosectioned, and stained. Compared with the scrambled control, the QKI-7 knockdown group showed significantly higher expression of EC marker CD144 along with QKI-7 suppression (pvalues: 0.0072, 0.0056) (e). GFP staining clearly shown that the Lentiviral constructs tagged with GFP targeted ECs in vivo (e). Scale bar:a200 μm;d100 μm;e200 μm. Data are from three biologically independent experiments. Error bars represent mean ± SEM (n= 3).Pvalues are shown: **p< 0.01, ns: not significant (two-tailedttest). Source data are provided as a Source data file. The formation of tube structures was observed at 6 and 8 h, which was quantified as tube length and meshed area using Image J. Cell barrier examination iPS-ECs were seeded on type IV mouse collagen (5 μg/ml; R&D Systems 3410-010-01)-coated E-Plate VIEW 16 (ACEA Biosciences, Inc. 300600890) in EGM-2 medium containing 25 ng/ml VEGF at 40,000 cells/well. Continuous monitor was performed overnight using xCELLigence RTCA DP (ACEA Biosciences, Inc.) in a standard CO 2 cell culture incubator until the cell index (CI) reached plateau, which represented the impedance of electron flow caused by adherent ECs. At this stage, the culture medium was replaced by OptiMEM to starve the cells for 2 h. Culture medium was subsequently changed to normal EGM-2 supplemented with 50 ng/ml VEGF and real-time CI monitoring continued for 24 h. In vivo Matrigel plug assay Animals used in these studies were housed with free access to standard food and water at a room temperature of 21 ± 2 °C relative humidity of 45 ± 15% and a 12-h-light/dark cycle. All experiments were performed in accordance with the Guidance on the Operation of the Animals (Scientific Procedures) Act, 1986 and approved by the Queen’s University Belfast Animal Welfare and Ethical Review Body. Work was performed under the project license number PPL2821. In total, 5 × 10 5 QKI-7-overexpressing iPS-ECs or control cells (iPS-ECs overexpressing an empty vector) were mixed with 150 µl Matrigel and injected subcutaneously into the back or flank of 10-week-old male C57BL/6 mice. Six injections were conducted for each group based on n = 3 biological replicates. Seven days later, the mice were sacrificed and the plugs were harvested and frozen in liquid nitrogen for cryosectioning and immunostaining. Nine plugs for each group were used for quantification. THP-1 adhesion In total, 2 × 10 4 iPS-ECs were seeded into wells of a 96-well plate and cultured at 37 °C in 5% CO 2 and 95% air humidified atmosphere. After 24 h, 1 × 10 4 Vybrant-labeled THP-1 cells were added into each well and co-cultured with iPS-ECs for 1 h. Thereafter, the cells were washed three times with PBS to remove the THP-1 cells in suspension. THP-1 adhesion was measured at six different areas under the microscope and the results were expressed as the number of THP-1 cells per mm 2 . Streptozocin (STZ)-induced diabetes in mice About 10 mg/ml STZ solution was prepared with citrate buffer at pH 4.5. Ten-week-old male C57BL/6 mice weighing more than 20 g were fasted for 4 h before intraperitoneal injection of STZ solution at 50 mg/kg (5 µl/g). Injections were performed for 5 consecutive days. One week later the blood glucose level was determined. Blood readings above 15 mmol/l were considered diabetic. All experiments were performed in accordance with the Guidance on the Operation of the Animals (Scientific Procedures) Act, 1986 and approved by the Queen’s University Belfast Animal Welfare and Ethical Review Body. Work was performed under the project license number PPL2821. Generation of shQKI-7 vector (pLV[miR30-shRNA]-Cd144>EGFP) shQKI-7 and shNT vectors under the CD144 promoter were designed for use in the in vivo experiments to target QKI-7 in ECs. shRNA sequence can only be driven by polymerase III promoters such as the U6 or H1 promoters. Since the tissue-specific promoter is a Pol II promoter, shRNA transcription was achieved via the miR30-based method, in which shRNA was embedded in a miR30 scaffold to be transcribed as an artificial miRNA expressing cassette. Vector ID VB180427-1084hrb. Experimental hindlimb ischemia The mouse hindlimb ischemia model was performed by ligation of femoral artery [30] , [60] . For EC transplantation, QKI-7 overexpressing iPS-ECs or control cells were trypsinized and 1 × 10 6 cells in 100 µl PBS were injected intramuscularly into the adductors of ischemic animals. For in vivo lentivirus infection, 10 8 transducing units (TU shRNA lentivirus) (non-targeting (NT) or QKI-7 (pLV[miR30-shRNA]-Cd144>EGFP) in a construct containing CD144 promoter, to target ECs) in 100 µl PBS was injected intramuscularly into the adductors. Tissue blood flow of both legs was sequentially assessed by Laser Doppler imaging (moorLDL2-IR) at 7 and 14 days. All experiments were performed in accordance with the Guidance on the Operation of the Animals (Scientific Procedures) Act, 1986 and approved by the Queen’s University Belfast Animal Welfare and Ethical Review Body. Work was performed under the project license number PPL2821. HRP-DAB immunohistochemical staining of human arterial tissue Arterial tissue was isolated from patients with critical limb ischemia undergoing a lower-limb amputation. Patients age: 72.7+/−11.3, sex: males 87.4%, degree of atherosclerosis: ***. Arterial plaques were graded according to the Oxford grading system. All human arterial samples were obtained with informed consent and procedures were performed in accordance with institutional guidelines and the Declaration of Helsinki (Ethical reference: 14/NW/1062). The ethics application was approved by the NRES Committee North West - Lancaster and Manchester Metropolitan University Internal Ethics Approval Committee. Tissue was fixed in 4% paraformaldehyde/PBS, processed for wax embedding and cut into 7-µm sections. Immunohistochemical analysis was carried out using the QKI-7 antibody (as above), alongside a mouse non-immune IgG control, and developed using the DAB-peroxidase system (Vector Laboratories) followed by counterstaining with Mayer’s haematoxylin [61] , [62] . Sections were imaged using the Panoramic SCAN with Zeiss Plan-apochromat 20×/0.8 objective (3D Histotech/Laser2000, Ringstead, UK). Statistical analysis Biological replicates were performed in all the experiments with n = 3. Data are expressed as the mean ± SEM and were analyzed using GraphPad Prism 5 software with a two-tailed Student’s t test for two groups or ANOVA for more than two groups. A value of * p < 0.05, ** p < 0.01, *** p < 0.001 was considered significant. Reporting summary Further information on research design is available in the Nature Research Reporting Summary linked to this article.